Tuning the range and stability of multiple phenotypic states with coupled positive–negative feedback loops Positive feedback loops can produce multistability, resulting in different phenotypic states. However, many transcription networks contain counteracting positive and negative feedbacks. Here we explore the dynamics of an interlinked positive and negative feedback motif based on the galactose-uptake control system of Saccharomyces cerevisiae modified to make the strength of each feedback externally controllable. Our results show that although the positive feedback loop determines the range of bistability and the width of the regions where intermediate activation is possible, the transition rates between states are mostly sensitive to the negative feedback strength. Thus, our results suggest that the function of the negative loop in this motif is to allow separate tuning of the range and transition rates between phenotypic states. This could enhance fitness by allowing improved matching of the stochastic switching to the frequency of environmental changes. Genetic networks comprise interactions between different agents, often interconnected through autoregulation circuits (feedback loops). The dynamic properties of these networks lead to emergent behaviours such as bistable or multistable outputs, adaptive responses and persistent memory [1] , [2] , [3] . One fundamental question in biology is what constraints, imposed by natural selection, have led to the observed architectures of these gene regulatory networks? It has been suggested that cells can exploit the dynamic properties of these networks in their adaptive responses to changes in the environment and under stress conditions, potentially enhancing fitness [4] , [5] , [6] , [7] , [8] , [9] , [10] , [11] , [12] , [13] , [14] . However, it is not clear which are the essential circuit features that provide control over this behaviour. The presence of positive feedbacks has been identified in several biological systems as a key regulatory motif in switching between stable states or in the generation of hysteresis [5] , [6] , [7] , [8] , [12] . Although it is well known that a single positive feedback, under appropriate conditions, is sufficient to generate a bistable switch in gene expression [5] , [6] , [7] , [8] , theoretical studies have suggested that the switching rates between these stable states cannot be independently tuned, and are restricted to the operating range of the positive feedback switch [15] . This limits the dynamic range and adaptability of the system. Many biological networks do not appear as single feedback loops. Instead, they present an interlinked pair of positive and negative feedback loops. An opposite positive–negative feedback motif may seem counterintuitive in that the added effects of the loops would appear to cancel each other out. However, this counteracting motif has been shown to be necessary to tune the dynamic aspects of a cell population. Of particular interest are the results of Tsai et al. [16] on the cell cycle of Xenopus oocytes. In these cells, a single delayed negative feedback was shown to be sufficient for providing the oscillations required to guide the cell cycle, making the presence of a positive feedback in this circuit apparently unnecessary. Upon further analysis, this positive feedback was found to provide cells with the ability to change the frequency of the oscillations independently of the amplitude, allowing for evolutionary tuning. These results point to the coupled-loop motif as a mechanism for providing tunability in multistable systems. Moreover, negative feedback regulation is not necessary to generate multistability, but it has been suggested to provide a mechanism for noise regulation [3] , [4] , [5] , [6] , [7] , [8] , [9] , [10] , [12] . In line with this, recent theoretical studies on toy models have suggested that a negative feedback may provide the ability to tune the frequency of switching between stable states [15] . This could be advantageous for a cell population needing to adjust to its environment, tuning its multistability range to the surrounding biochemical parameters and adjusting its switching rates to match the rates of environmental changes and the constraints imposed by genetic noise. Therefore, a properly tuned positive–negative feedback motif may be sufficient to accomplish the required tuning necessary for cell population adaptation to environmental conditions and fluctuations. An example of a coupled positive and negative feedback motif is the galactose uptake network of Saccharomyces cerevisiae. Extensive research has elucidated a detailed map of the molecular interactions that comprise the feedback network [17] , [18] , [19] , [20] , [21] , [22] ( Supplementary Fig. S1 ). This network is a good example of an autoregulatory genetic circuit, containing an interlinked positive and negative feedback loop through Gal3p and Gal80p proteins, respectively ( Fig. 1a ). In the present work, we illustrate the regulatory capacity of this interlinked positive–negative feedback motif experimentally by re-engineering the galactose uptake system in such a way that the strength of either feedback can be externally controlled. We investigate how the strength of each feedback loop inside this motif affects the systems properties, including the range of bimodality and the transition rates between phenotypic states, and show that noise is modulated differently by each loop. 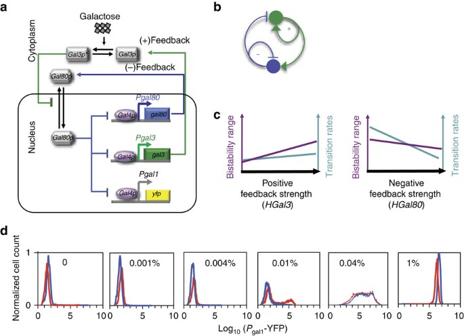Figure 1: The GAL system inS. cerevisiae. (a) This system controls the uptake machinery for galactose: extracellular galactose is imported into the cell promoting the transcriptional activation of thegalgenes. Key features include a negative feedback loop (blue line) in which Gal80p inhibits expression of thegalgenes and a positive feedback via Gal3p (green line). (b) Sketch of the interlinked positive and negative feedback loops in the core galactose uptake system. (c) Sketch of the expected effects of varying the strength of each feedback on the region of bistability and transition rates (Supplementary Fig. S4). (d) Wild-type protein expression distributions obtained by flow cytometry using the reporter protein YFP under the control of thegal1promoter (Pgal1). Blue and red distributions denote cells that were initially grown for 12 h without galactose (but with 2% of glucose (non-induced)) and with 2% of galactose and 0.02% of glucose (fully induced), respectively. After this period, cells were grown for a further 30 h in different concentrations of galactose as specified. Figure 1: The GAL system in S. cerevisiae . ( a ) This system controls the uptake machinery for galactose: extracellular galactose is imported into the cell promoting the transcriptional activation of the gal genes. Key features include a negative feedback loop (blue line) in which Gal80p inhibits expression of the gal genes and a positive feedback via Gal3p (green line). ( b ) Sketch of the interlinked positive and negative feedback loops in the core galactose uptake system. ( c ) Sketch of the expected effects of varying the strength of each feedback on the region of bistability and transition rates ( Supplementary Fig. S4 ). ( d ) Wild-type protein expression distributions obtained by flow cytometry using the reporter protein YFP under the control of the gal1 promoter (P gal1 ). Blue and red distributions denote cells that were initially grown for 12 h without galactose (but with 2% of glucose (non-induced)) and with 2% of galactose and 0.02% of glucose (fully induced), respectively. After this period, cells were grown for a further 30 h in different concentrations of galactose as specified. Full size image The wild-type strain displays noisy multistability We used the galactose uptake network in S. cerevisiae (GAL system) as a model for a positive–negative feedback motif. The galactose uptake regulatory network functions as follows ( Fig. 1a ): when galactose is absent, Gal80p inhibits the function of Gal4p, which is a constitutively bound transcriptional activator of the GAL genes [17] , [18] , [19] , [20] , [21] , [22] . In the presence of intracellular galactose, the sugar binds to the protein Gal3p, resulting in its activation. This active complex Gal3p–Galactose then binds and sequesters the cytoplasmatic Gal80p protein, depleting Gal80p from the nucleus [19] . Gal4p is then released from the inhibitory action of Gal80p, activating the expression of the GAL genes [18] ( Fig. 1a ). Thus, the loop through Gal80p provides a negative feedback, whereas the loop through Gal3p provides a positive feedback ( Fig. 1a ). The GAL network includes other inputs such as gal2 and gal1 , but these do not appear to fundamentally change the behaviour of the system [1] . We examine the GAL system by obtaining the distributions of protein expression levels in a population of cells using flow cytometry. For high and low concentrations of galactose, the population shows a narrow distribution around a high (ON) and low (OFF) expression level, respectively. For intermediate concentrations, the wild-type system can have a bimodal or broad distribution. Previous studies [1] have shown that if the negative feedback loop is knocked out, at intermediate concentrations of galactose the system can show hysteresis (memory) for long periods, where the distribution will be ON or OFF depending on its previous history. These two distribution types provide contrasting advantages for a cell population. The hysteretic distribution would allow for a population of cells to persist in an ON state in the presence of fluctuations of a food source, therefore sparing the metabolic cost of reinitiating the synthesis of the uptake machinery after a transient fluctuation. The broad distribution would allow for bet-hedging and for anticipation of a long-term switching of available food sources [13] . The concentrations in which it would be advantageous for a cell to be in any of those states will depend on biochemical details, such as the metabolic cost of producing the enzymes and the amount of energy that can be obtained from the sugar. We will refer to the range of concentration where a cell exhibits hysteresis or a bimodal or broad distribution as the range of bistability. Cells within a bimodal distribution do not stay at a particular level of expression; even if the distribution is at a steady state, cells will be transitioning between high- and low-expression levels due to the inherent stochasticity in gene expression [23] . This effect complicates analytical modelling: for parameters where a deterministic model [15] shows hysteresis, a Monte-Carlo simulation [24] can show bimodality. Furthermore, the transition rates determine the type of distribution: slow transitions result in memory and fast transitions result in a broad distribution. It has been shown [13] that the switching rate must match the rate of changes in the environment for the cell to have a selective advantage, and that the rate can be changed by knocking out the negative feedback loop. The dependence of the range of bistability and the switching rates on the feedback loops can be tested on the stochastic simulations of the basic model [15] , which suggest that the range of bistability depends primarily on the strength of the positive feedback loop, whereas the transition rates between the two stable states within the broad region seem markedly sensitive only to the strength of the negative feedback, as depicted qualitatively in Fig. 1c . To test this experimentally, we measured the distribution of expression for a wild-type circuit and two versions where the strength of the feedbacks could be externally tuned, for different concentrations of galactose in populations that had been previously forced to have low expression (OFF history) or high expression (ON history). This was done by initially placing the wild-type strain in either the ON or OFF conditions by growing the cells for 12 h in media with 2% galactose or 2% glucose (an alternative carbon source), respectively ( Supplementary Fig. S2 ). Subsequently, cells from these preparation media are transferred into varying concentrations of galactose and allowed to grow for 30 h. This incubation time ensures that the population distributions have reached a steady state and are no longer changing quickly. Throughout the experiments, cells were grown at low densities to ensure that galactose depletion is negligible [1] (see Methods section) and glucose is used as a background carbon source. As the GAL genes can be repressed by glucose [17] , we maintained a low-enough concentration of this sugar to ensure that the system does not show significant variations as the galactose concentration is changed ( Supplementary Fig. S3 and see Methods section). The resulting histograms of the wild-type GAL expression levels (measured by flow cytometry) after exposure to a series of galactose concentrations are shown in Fig. 1d . The histograms are colour coded to indicate that the system initiated in an ON (red) or OFF (blue) state. After 30 h, at low (<0.01%) and high (>0.04%) galactose concentrations, the protein expression distributions approach the same unique ON or OFF distributions, respectively, indicating monostability. At a galactose concentration of 0.04%, protein levels present a broad distribution in gene expression that ranges between the ON and OFF states but show no memory, whereas at 0.01% the system is mostly OFF for both initial states but shows a slight bimodality (and, therefore, some memory) for the initially ON population. The feedback strength determines the cell’s phenotype To change the strength of the feedbacks, two haploid strains were constructed in which the g al3 or gal80 promoter regions of the galactose circuit were re-engineered using a dual system in which the reverse tetracycline controlled transactivator and a tetracycline-inactivable tTA-Ssn6 repressor coexist in the same cell [25] . As in the wild-type strain, the network activity in single cells was monitored by flow cytometry through the expression of yeast fluorescent protein (YFP) driven by the gal1 promoter. The implementation of this dual system reduces basal expression of the Ptet promoter in the absence of doxycycline, allowing us to achieve a tighter regulation of gene expression ( Supplementary Fig. S5 ) [25] . With these modifications, it is possible to modulate the strength of each feedback motif (defined as autosensitivity) by changing the concentration of doxycycline while maintaining a multiloop architecture (see Supplementary Note 1 ). In Fig. 2c,d , the dynamic behaviour of each rewired circuit is mapped over a broad range of galactose and doxycycline concentrations. In these maps, the colour codes reflect the distribution phenotypes shown in Fig. 2b (see Supplementary Fig. S6 and Supplementary Note 2 ). We observe that when the negative feedback strength is varied over a broad range of galactose/doxycycline concentrations, the system displays monostable ON and OFF regions (green and blue, Fig. 2c ), separating an ON/OFF transition regime displaying a broad distribution of phenotypes (orange, Fig. 2c ). The positive-feedback strength map ( Fig. 2d ) also displays monostable ON and OFF regions, and a ‘broad’ distribution region, but also a region of hysteresis or epigenetic ‘memory’, where cells that are first grown at a high galactose concentration maintain their phenotypic ON state when transferred to intermediate concentrations and cells that are first grown at a low galactose concentration maintain their phenotypic OFF state when transferred to intermediate concentrations. These results clearly show that feedback strength determines the phenotypic behaviour of the cell populations, modulating the range of different stable states. Variations in feedback strength allow the system to access, first, to regions of high cell variability in the case of the negative feedback modulation and, second, to regions of epigenetic memory in the case of the positive feedback modulation. It is noteworthy that in both cases, the wild-type is poised at the edge of the region where the OFF state disappears. 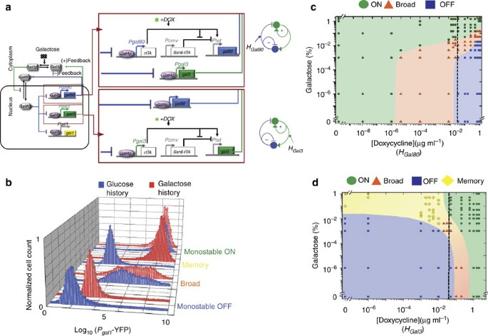Figure 2: Accessing different expression phenotypes through the regulation of the feedback strengths. (a) To test the effects of independent modulation of the positive and negative feedbacks, two different strains were constructed, where (i) the negative feedback strength is controlled externally leaving the positive feedback unaltered, and (ii) the positive feedback strength is controlled externally leaving the negative feedback unaltered. The circuit was modified to express thegal80orgal3genes from a tetracycline-inducible promoter (Ptet), and to reclose the loops the expression of reverse tetracycline controlled transactivator (rtTA) protein was placed under the control of the promotergal80orgal3. In addition, to reduce basal expression of the Ptetpromoter in absence of doxycycline, we inserted in both circuits the tetR-Ssn6 repressor system (Supplementary Fig. S5). The activity of the pathway was read out using the reporter protein YFP under the control of thegal1promoter. (b) YFP fluorescence distributions for different galactose concentrations and different feedback loop strengths. These distributions are grouped as ON (Green), OFF (Blue), memory (Yellow) or broad (Orange;Supplementary Fig. S6andSupplementary Note 2). ‘Broad’ here refers to wide distributions with averages at intermediate values of expression between the ON and OFF states. The distribution phenotypes are mapped as a function of galactose external concentration and feedback strength for (c) negative feedback and (d) positive feedback. The dashed line represents the approximate range of expression equivalent to wild type in each system as identified by flow cytometry (Fig. 1d) and mRNA FISH. Figure 2: Accessing different expression phenotypes through the regulation of the feedback strengths. ( a ) To test the effects of independent modulation of the positive and negative feedbacks, two different strains were constructed, where (i) the negative feedback strength is controlled externally leaving the positive feedback unaltered, and (ii) the positive feedback strength is controlled externally leaving the negative feedback unaltered. The circuit was modified to express the gal80 or gal3 genes from a tetracycline-inducible promoter (P tet ), and to reclose the loops the expression of reverse tetracycline controlled transactivator (rtTA) protein was placed under the control of the promoter gal80 or gal3 . In addition, to reduce basal expression of the P tet promoter in absence of doxycycline, we inserted in both circuits the tetR-Ssn6 repressor system ( Supplementary Fig. S5 ). The activity of the pathway was read out using the reporter protein YFP under the control of the gal1 promoter. ( b ) YFP fluorescence distributions for different galactose concentrations and different feedback loop strengths. These distributions are grouped as ON (Green), OFF (Blue), memory (Yellow) or broad (Orange; Supplementary Fig. S6 and Supplementary Note 2 ). ‘Broad’ here refers to wide distributions with averages at intermediate values of expression between the ON and OFF states. The distribution phenotypes are mapped as a function of galactose external concentration and feedback strength for ( c ) negative feedback and ( d ) positive feedback. The dashed line represents the approximate range of expression equivalent to wild type in each system as identified by flow cytometry ( Fig. 1d ) and mRNA FISH. Full size image Transition rates respond to negative feedback strength The protein distribution is expected to be ‘broad’ when there is a high level of noise, and the system would then be governed by high transition rates between what would be stable states in the deterministic model. In the presence of changes in external conditions, such as a sudden change in galactose concentration, this phenotype would be characterized by fast equilibration rates into a new state. On the other hand, the persistent memory phenotype would be characterized by having low equilibration rates. To test this prediction experimentally, we monitored the rate of relaxation from a monostable distribution state (either ON or OFF) into either a broad distribution state ( Fig. 3a ) or a hysteretic distribution state ( Fig. 3b ) for the strain with the perturbed positive feedback. As expected, the equilibration rates are faster when the final state is a broad distribution than when the end state is a hysteretic distribution ( Fig. 3a,b ). This also means that equilibration rates in the bimodal region depend on the strength of the positive feedback, as predicted by Pfeuty and Kaneko [15] . However, as the wild-type system does not operate in this region, but in one where the transitions for different galactose levels go from OFF to ‘broad’ to ON ( Fig. 2c,d ), we assessed how the positive and negative feedback strengths influenced the dynamic behaviour in this region. For this, we measured the equilibration rates from the ON and OFF states to different final states within the broad region. This corresponds to tuning each of the feedback strengths through changes in doxycycline concentration while maintaining the galactose concentration constant so that changes in the dynamic behaviour induced by variations in galactose are excluded. The transition into the intermediate state is measured by plotting the fraction of ON cells as a function of time. This is then modelled as a two-state system evolving towards their equilibrium. 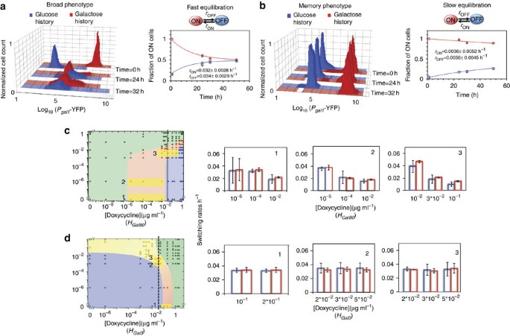Figure 3: Modulation of negative feedback strength defines the presence or absence of long-term memory. YFP fluorescence distributions are measured at different time points after transferring cells from an all-on (red) or an all-off (blue) state into intermediate galactose and doxycycline concentrations. The transition into the intermediate state is measured by plotting the fraction of ON cells as a function of time. Transition rates are obtained by fitting the data as described in the main text (dashed lines). As expected, transition rates are higher for the broad phenotype (a) compared with the memory phenotype (b) for the strain with the perturbed positive feedback. The transition rates are plotted as a function of the negative (c) and the positive (d) feedback loop strengths for different trajectories (1, 2, 3) inside the broad phenotypic state region, showing that the transition rates are only sensitive to the negative feedback strength. Results are expressed as mean (+s.e.m.) of at least three independent experiments. Transition rates are obtained by fitting the data with the function Figure 3: Modulation of negative feedback strength defines the presence or absence of long-term memory. YFP fluorescence distributions are measured at different time points after transferring cells from an all-on (red) or an all-off (blue) state into intermediate galactose and doxycycline concentrations. The transition into the intermediate state is measured by plotting the fraction of ON cells as a function of time. Transition rates are obtained by fitting the data as described in the main text (dashed lines). As expected, transition rates are higher for the broad phenotype ( a ) compared with the memory phenotype ( b ) for the strain with the perturbed positive feedback. The transition rates are plotted as a function of the negative ( c ) and the positive ( d ) feedback loop strengths for different trajectories (1, 2, 3) inside the broad phenotypic state region, showing that the transition rates are only sensitive to the negative feedback strength. Results are expressed as mean (+s.e.m.) of at least three independent experiments. Full size image and minimizing the χ 2 -cost function ( Fig. 3 ). For the doxycycline concentrations evaluated, we observe that increasing the strength of the negative feedback loop decreases the switching rates independently of the galactose concentration ( Fig. 3c ). In contrast, increasing the positive feedback strength does not have a significant effect on the transition rates ( Fig. 3d ). Therefore, although the positive feedback with ultrasensitivity is sufficient for generating multistability, it does not appear to modulate the transition rates between different phenotypic states in the broad area. In contrast, the negative feedback presents a suitable motif that allows the system to regulate these transitions. This is consistent with the expected results sketched in Fig. 1c , which show that the transition rates respond to changes in the negative feedback strength but not to changes in the positive feedback strength. Feedback loops regulate effects of different noise sources From a deterministic view, positive and negative feedbacks would be expected to partially cancel each other out as the relative strength of the two feedback loops would determine the height of the equivalent potential barrier that separates stable states. If equilibration rates depended only on the height of these equivalent potential barriers [1] , the equilibration rates would be equally sensitive to both feedback strengths. From a stochastic point of view, not only the potential barriers but also the amount of fluctuations are influenced by the feedbacks. Previous theoretical work suggests that the main source of noise is the variability in the mRNA copy number related to promoter fluctuations [23] , [26] . This previous work showed that the mRNA copy number noise would, in principle, be amplified by the positive feedback and dampened by the negative feedback. However, fluctuations in the number of gal3 or gal80 mRNAs can come both from the intrinsically random nature of gene expression (intrinsic fluctuations) and from the transmitted fluctuations from the regulators of expression and variations in global factors (extrinsic fluctuations) [2] , [23] , [27] , [28] , [29] , [30] , making the prediction of mRNA copy-number noise non-trivial. To investigate this further, we determined the relative contributions of each of these two noise sources as a function of feedback strength. We counted the number of both endogenous gal3 and gal80 mRNA molecules in individual cells that have been fixed at a given feedback strength using mRNA fluorescence in situ hybridization (FISH) ( Fig. 4 ) [27] , [31] . As the extrinsic noise affects both genes simultaneously, correlated variation in mRNA numbers indicates that the primary noise source is extrinsic, whereas uncorrelated variations indicate an intrinsic origin for mRNA fluctuations [32] . We observe that in the strain with tunable negative feedback the numbers of mRNA molecules of the two genes are mostly uncorrelated, indicating the prevalence of intrinsic noise. In contrast, in the strain with tunable positive feedback the correlation between genes is high, except for low-feedback strengths ( Fig. 4d,e ). Although this in itself does not elucidate the mechanism for the difference in the sensitivity of the transition rates to the feedback strengths, it does indicate that the different modulation of the noise by each loop might have a role. 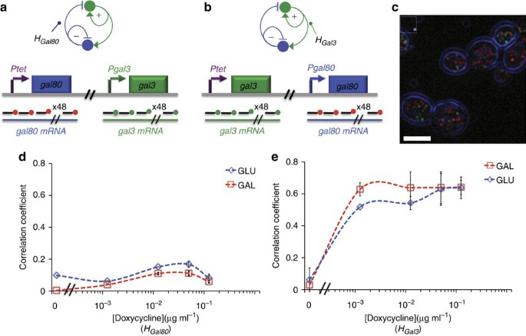Figure 4: Noise levels are modulated independently by each feedback motif. (a,b) Detection of single mRNA molecules (gal3andgal80) by FISH in the strains in which the feedback loops were perturbed. Multiple specific fluorescent probes bind to each mRNA molecule (gal3(green) orgal80(red)), yielding distinct fluorescent signals. As the stochastic expression of genes can depend on the positioning of the genes along the chromosomes36, the chromosomal position of the genesgal3 andgal80 in the modified strains is similar to that of the wild-type system. (c) Pseudo-coloured fluorescent image, in which thegal3gene was hybridized to 48 FISH probes (Cy5) that bind to thegal3open-reading frame (ORF) and thegal80gene was hybridized to 48 FISH probes (Alexa 594) that bind to thegal80ORF. Dots correspond to individual mRNA molecules. Scale bar, 5 μm. (d,e). Correlation coefficients are plotted as a function of the strength of the feedback loops, for negative (d) and positive (e) feedback loops (Supplementary Fig. S7). Blue and red points denote cells that were initially grown for 12 h in 0% galactose and 2% glucose, and in 2% galactose and 0.02% glucose, respectively. After this period, cells were grown for a further 30 h in the specified doxycycline concentrations. Results are expressed as mean (+s.e.m.) of at least three independent experiments. Figure 4: Noise levels are modulated independently by each feedback motif. ( a , b ) Detection of single mRNA molecules ( gal3 and gal80 ) by FISH in the strains in which the feedback loops were perturbed. Multiple specific fluorescent probes bind to each mRNA molecule ( gal3 (green) or gal80 (red)), yielding distinct fluorescent signals. As the stochastic expression of genes can depend on the positioning of the genes along the chromosomes [36] , the chromosomal position of the genes gal 3 and gal 80 in the modified strains is similar to that of the wild-type system. ( c ) Pseudo-coloured fluorescent image, in which the gal3 gene was hybridized to 48 FISH probes (Cy5) that bind to the gal3 open-reading frame (ORF) and the gal80 gene was hybridized to 48 FISH probes (Alexa 594) that bind to the gal80 ORF. Dots correspond to individual mRNA molecules. Scale bar, 5 μm. ( d , e ). Correlation coefficients are plotted as a function of the strength of the feedback loops, for negative ( d ) and positive ( e ) feedback loops ( Supplementary Fig. S7 ). Blue and red points denote cells that were initially grown for 12 h in 0% galactose and 2% glucose, and in 2% galactose and 0.02% glucose, respectively. After this period, cells were grown for a further 30 h in the specified doxycycline concentrations. Results are expressed as mean (+s.e.m.) of at least three independent experiments. Full size image In summary, our results show that modulation of the positive and negative feedback in this coupled motif determines the phenotypic behaviour of the cell populations, modulating both the range of external conditions where different expression states are possible and the stability of such states. We suggest that although only the positive feedback is required for generating multistability in response to induction, it is not sufficient for independent regulation of the transition rates between different phenotypic states. Within the biologically relevant regime for this strain, this fine-tuning is only possible through the presence of the negative feedback. One of the basic functions of genetic networks is to activate certain genes in response to an external stimulus. The fitness conferred by such a circuit depends on how well its response matches with the optimal response defined by the biochemical parameters. For a metabolic switch, this means turning the circuit ON, OFF, or having a certain distribution of activation levels at a given external input. The presence of a single positive feedback is sufficient to achieve this. However, this level of flexibility may not be sufficient to optimize the system. A recent study has shown that cells that tune interphenotype switching rates to the frequency of environmental fluctuations [13] present a fitness advantage. In the GAL system, this implies that cells not only have to adjust the circuit to be able to switch at a specific concentration of galactose but also have to match their switching rates to how often the external galactose concentration changes. These would be two constraints that need to be modulated independently. We show that the presence of the negative feedback allows separate tuning of the switching rates, possibly by modulating the intrinsic fluctuations of the system. This would provide the evolution process with two knobs to play with, allowing for separately optimizing the switching threshold to the biochemical parameters and the switching rate to the level of fluctuations in the environment based on the interlinked feedback motif. The frequent presence of interlinked positive and negative feedback loops in natural biological networks suggests that this type of design possesses some performance advantages over single positive feedback loops, and the present work demonstrates that this coupled loop design provides the ability to tune both the range of conditions where different phenotypic states are possible and the switching rates between these states. Strain background and construction A list of strains with a complete description is provided in the Supplementary Information . All strains were derived from the haploid strain of S. cerevisiae W303 ( MATα , his3::HIS3/his3 and ade2/ade2::ADE2-P gal1 -YFP ) referred to as the ‘wild type’ in our study. The native P gal1 , P gal3 and P gal80 promoters, as well as the gal3 and gal80 genes, were amplified from the wild-type strain by PCR using Pfx DNA polymerase (Invitrogen). The P gal1 , P gal3 and P gal80 promoter sequences correspond to 669, 830 and 632 bp regions upstream of the start codon of the respective genes. These sequences include all the known binding sites of transcription factors for the respective genes [1] . Promoter–protein constructs were generated using standard PCR and enzyme restrictions techniques, and cloned into S. cerevisiae integration vectors pRS402 and pRS306 (EUROSCARF). Correct disruptions of the strains genes were done with PCR-generated kanMX molecules (PUG6 vector) flanked by 50 bp of the yeast homologous DNA at either side. Wild-type strain was transformed with the resulting constructs by using the LiAc yeast transformation procedure [33] . Construct integration into the chromosome was verified in all cases by PCR. To attenuate leakiness in the expression of the target genes by the P teto2 promoter in absence of doxycycline, a dual system in which the tetO -binding activator and a tetO -binding repressor (both of them regulated by tetracycline in opposite ways) coexist in the same cell was used. This implementation permits to achieve a tighter regulation of gene expression ( Supplementary Fig. S5 ) [25] . Flow cytometry For the history period, cells were grown overnight at 30 °C in yeast nitrogen base media with the appropriate amino-acid supplement (complete supplement mixture) and 0.02% glucose as a background carbon source. Media used for fully induced history experiments (ON) were supplemented with 2% galactose, whereas media for non-induced experiments (OFF) contained 2% glucose as the sole carbon source. In addition to lock the cells from the strain MSY019 into the OFF state, 0.1 μg ml −1 of doxycycline was added to the media. The same amount of doxycycline was added to the media to lock cells from the strain MSY020 into the ON state. The distributions in steady state for this history period are show in the Supplementary Fig. S2 . After this history period, cells were spun down, washed and resuspended in yeast nitrogen base media with the appropriate amino-acid supplement (CSM), 0.02% glucose and various concentrations of galactose and doxycycline. For this induction period, cells were diluted to an OD 600 value so that after 30 h of growth the galactose and glucose concentration in the medium would not change by more than 10% (final OD 600 0.05). Cells were grown at 30 °C. After the induction period of 30 h, the expression distributions were determined by flow cytometer (FACScan; Becton Dickinson). To determine that nutrients in the media are not being depleted after the induction period, it is possible to calculate the depletion of sugars during exponential growth over time according to the following equation [34] : In which r is the uptake rate per A 600 nm , measured in units of mM h −1 A 600 nm −1 . N(t)−N(0) is the change in A 600 nm of the cells measured using the spectrophotometer (Hitachi U-1800) and μ is the growth rate. For glucose, we have the glucose uptake rate for S. cerevisiae [34] is 1.2 mM h −1 A 600 nm −1 . The A 600 nm after the induction period was 0.05 and at the beginning was 10 −7 . The growth rate determined for our strains in glucose is 0.37 h −1 . Therefore, we have that the glucose depletion after the induction period follows: If the initial concentration of glucose is 0.02%, according to the previous result after 30 h the amount that is available is 0.017%. Therefore, just 16% of the initial amount is consumed. The same analysis can be done for galactose by using an uptake rate [1] of 0.084 mM h −1 A 600 nm −1 and the growth rate determined for our strains in galactose, which is 0.3 h −1 . In this case, not even 10% of the initial amount is consumed, as reported previously [1] . Data analysis Cells were analysed by flow cytometry based on scattered laser light and fluorescence from a focused 488-nm argon ion laser. The data for each event consisted of the forward light scatter (FSC), perpendicular light scatter (SSC), pulse width of the forward scattered light and the integrated fluorescence to quantify the YFP concentration. Data from a single run of the flow cytometer were stored in a Flow Cytometry Standard format file incorporating 15,000 events in a specific gate. Initial visualization of the flow cytometry data was performed using MFI software and then analysed using Matlab (Mathworks, Natick, MA). For each data point, we recorded the number of events and computed the average and s.d. of the fluorescence intensity. To select events with homogeneous cell size and avoid fluorescence variation coming from cell size variation, we selected events within a gate of forward light scatter (FSC) based on the mean FSC±0.1 s.d. of the FSC of the control strain. Mutant and wild-type data were gated with the same FLS window size to avoid introducing bias. RNA FISH experiment For the FISH experiments, cells were grown as described in the flow cytometry section. After induction period, yeast cultures were fixed with formaldehyde for 40 min at room temperature with gentle rocking throughout. Zymolyase digestions were performed at 30 °C in 0.5 ml buffer B containing 2 mg ml −1 Zymolase 100T (US Biological) for 15 min while rotating tubes. Hybridizations with DNA probes were performed in 10% formamide hybridization buffer. gal80-specific probes were coupled to Alexa-594 (Invitrogen) and gal3-specific probes were coupled to Cy5 (GE Amersham). To protect fluorophores from oxidation during imaging, cells were suspended in GLOX buffer and imaged on Lab-Tek II chambered coverglass (Thermo Fisher Scientific, Billerica, MA) previously incubated with ConA at 0.1 ng ml −1 (Sigma Aldrich, St Louis, MO). Probes for in situ hybridization The gal3 and gal80 mRNA were each labelled with a unique set of up to 48 DNA oligonucleotides, each with a length of 20 nt. The 3′-end of each probe was modified with an amine group. The DNA probes have been coupled to Alexa fluor 594 or Cy5. After coupling the DNA probes to the fluorophore, the probes were ethanol precipitated and were purified on an HPLC column to isolate oligonucleotides displaying the highest degree of coupling of the fluorophore to the amine groups. Fluorescence microscopy image acquisition and analysis Images were collected using a Nikon TE2000 inverted fluorescence microscope with 1,003 oil-immersion objective, appropriate filters (Alexa594, Cy5 and DAPI (4′,6-diamidino-2-phenylindole)) and a Princeton Instruments camera with MetaMorph software (Molecular Devices, Downington, PA). Custom filter sets were designed to distinguish Alexa594 and Cy5 signal. Differential interference contrast (DIC), DAPI, Alexa594 and Cy5 images were collected with 0.2-μm z -slices. Analysis was done as described previously [35] . In general, DIC and DAPI images were used to identify individual cells. Alexa594 and Cy5 image stacks were used to detect RNA transcripts. For image processing, a DIC image was chosen in which a clear cell boundary could be observed. This image was converted into a binary image using automated thresholding. The maximum projection of a DAPI image stack was generated and converted into a binary image using a fixed pixel intensity threshold. The binary DIC image was merged with the binary DAPI image. DAPI-stained nuclei were used in running a marker-controlled watershed algorithm over the merged DIC/DAPI image. Cell boundaries of individual cells were obtained using an edge-detection algorithm. Connected regions measuring larger than the expected range of sizes for an individual cell were rejected. The number of RNA transcripts in each cell was counted using a programme that operates as follows: to enhance particulate signals, the programme runs a median filter followed by a Laplacian filter on each optical slice. A threshold was then selected to detect individual dots in each plane. The particle count was robust over a range of selected thresholds. Images that demarcated cell boundaries were merged with each plane of Alexa594 or Cy5 image stacks. This processing enabled the programme to count the total number of isolated signals in three dimensions within each cell. Simulations Model predictions were generated by Monte-Carlo simulation by implementation of a modified Gillespie’s stochastic simulation algorithm [24] in Matlab (MathWorks). How to cite this article: Avendaño, M. S. et al. Tuning the range and stability of multiple phenotypic states with coupled positive–negative feedback loops. Nat. Commun. 4:2605 doi: 10.1038/ncomms3605 (2013).